Prions disturb post-Golgi trafficking of membrane proteins Conformational conversion of normal cellular prion protein PrP C into pathogenic PrP Sc is central to the pathogenesis of prion diseases. However, the pathogenic mechanism remains unknown. Here we show that post-Golgi vesicular trafficking is significantly delayed in prion-infected N2a cells. Accordingly, cell surface expression of membrane proteins examined, including PrP C , insulin receptor involved in neuroprotection, and attractin, whose mutation causes prion disease-like spongiform neurodegeneration, is reduced. Instead, they accumulate in the Golgi apparatus. PrP Sc is detected throughout endosomal compartments, being particularly abundant in recycling endosome. We also show reduced surface expression of PrP C and insulin receptor in prion-infected mouse brains well before the onset of disease. These results suggest that prion infection might impair post-Golgi trafficking of membrane proteins to the cell surface in neurons via PrP Sc accumulated in recycling endosome, and eventually induce neuronal dysfunctions associated with prion diseases. The normal cellular prion protein, PrP C , is a glycosylphosphatidylinositol (GPI)-anchored membrane glycoprotein expressed most abundantly in neurons [1] . Conformational conversion of PrP C into the abnormally folded, relatively proteinase K (PK)-resistant PrP Sc has a pivotal role in prion diseases such as Creutzfeldt-Jakob disease and scrapie [1] . Mice devoid of PrP C ( Prnp 0/0 ) are resistant to prion disease even after intracerebral inoculation with prions [2] , [3] , [4] , [5] . However, the pathogenic mechanism of the diseases is unknown. The Golgi apparatus is a specialized cytoplasmic organelle near the nucleus that sorts membrane and luminal proteins via vesicle transport from the endoplasmic reticulum (ER) to lysosomes, secretory vesicles and the cell surface. In neurons, it is involved in the axonal transport of proteins, and functional damage to it could have significant implications. Indeed, the Golgi apparatus might have a role in various neurodegenerative disorders, including Alzheimer’s disease, Parkinson’s disease and amyotrophic lateral sclerosis [6] , [7] . Reports suggest involvement of the Golgi apparatus in prion diseases. PrP Sc has been detected near the Golgi apparatus in prion-infected cells [8] . Transgenic (tg) mice expressing PrP fused with green fluorescent protein on the wild-type background, that is, tg(PrP-EGFP)/ Prnp +/+ mice, developed prion disease after intracerebral inoculation with RML prions, with progressive accumulation of PrP-EGFP in the Golgi apparatus of neurons from the early stages of the infection [9] . The transmembrane form of PrP, Ctm PrP, with the N terminus in the cytosol and C terminus in the ER lumen is neurotoxic, causing prion disease-like neurodegeneration in mice [10] , [11] . Tg mice expressing a Ctm PrP-favouring mutant accumulated Ctm PrP at the Golgi apparatus in neurons [12] , [13] . Insulin signalling may regulate a neuroprotective function, synaptic plasticity and memory formation [14] , [15] , [16] , [17] , [18] , [19] , [20] , [21] . Loss-of-function for attractin causes prion disease-like spongiform neurodegeneration in animals [22] . However, the role of the insulin receptor (IR) and attractin in prion diseases is unknown. In the present study, we show that post-Golgi vesicular trafficking is delayed in mouse neuroblastoma N2a cells persistently infected with scrapie prions. PrP C cell surface expression diminishes and instead accumulates in the Golgi apparatus. Most PrP Sc is in endosomal compartments, being particularly abundant in recycling endosomes. We also show that cell surface IR and attractin are reduced in infected cells, and downstream signalling of the IR is disturbed. Furthermore, cell surface PrP C and IR are reduced in prion-infected mouse brains well before the onset of clinical symptoms. Another GPI-anchored membrane molecule, Thy-1, also reduces surface expression in infected brains. However, the glutamate receptor subunits GluR3 and NR1 are not affected. These results suggest that prion infection could impair post-Golgi vesicle transportation of some membrane proteins, including PrP C , Thy-1, IR and attractin, to the cell surface by accumulating PrP Sc in recycling endosomes eventually causing neuronal dysfunction. Post-Golgi trafficking is delayed in prion-infected cells Uninfected N2aC24 line is a cloned N2a line overexpressesing exogenously transfected mouse PrP C (ref. 23 ). Infected N2aC24L1-3 line is a clone of N2aC24 cells that were infected with 22L prions [23] . PrP Sc was detectable in infected N2aC24L1-3 cells on western blotting (WB) ( Fig. 1a ). Cured N2aC24L1-3 cells were established in this study. Prion infection was cured by treatment with SAF32 anti-PrP antibody (Ab) against the octapeptide repeat region. Cured N2aC24L1-3 cells lack PrP Sc ( Fig. 1a ). The Golgi apparatus is important for vesicular trafficking of membrane and secretory molecules. To assess the vesicular trafficking in these cells, we performed a vesicular transport assay with a temperature-sensitive mutant of the vesicular stomatitis virus-G protein fused with green fluorescent protein (GFP), designated VSV-G(ts045)–GFP. VSV-G(ts045)–GFP folds improperly at the non-permissive temperature of 39.5 °C, thereby remaining in the ER. In contrast, at the permissive temperature of 32 °C, the protein is properly folded and exits from the ER to the Golgi apparatus and then to the cell surface. 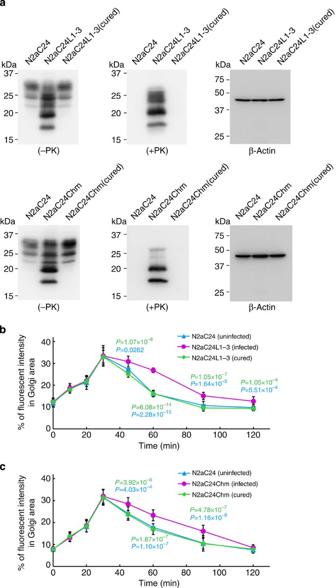Figure 1: Post-Golgi vesicular trafficking is delayed in 22L prion-infected N2aC24L1-3 and Chandler prion-infected N2aC24Chm cells. (a) Upper panels: WB of uninfected N2aC24, infected N2aC24L1-3 and cured N2aC24L1-3 cells with 6D11 anti-PrP Ab. Lower panels: WB of uninfected N2aC24, infected N2aC24Chm and cured N2aC24Chm cells with 6D11 anti-PrP Ab. PrPScwas detected in infected N2aC24L1-3 or N2aC24Chm cells, but not in uninfected N2aC24, cured N2aC24L1-3, and cured N2aC24Chm cells. Each cell lysate was treated without (−) or with (+) PK. β-Actin is an internal control. (b) Transport assay of VSV-G(ts045)–GFP in uninfected N2aC24, infected N2aC24L1-3 and cured N2aC24L1-3 cells. (c) Transport assay of VSV-G(ts045)–GFP in uninfected N2aC24, infected N2aC24Chm and cured N2aC24Chm cells. Cells were transfected with the vector encoding VSV-G(ts045)–GFP and incubated at the non-permissive temperature at 39.5 °C. Fluorescent intensities for VSV-G(ts045)–GFP at the Golgi region against those in the whole cell were determined in the randomly selected transfected cells (n=14–16) at various times, after the cells were transferred to the permissive temperature of 32 °C. Trafficking of VSV-G(ts045)–GFP in the cells was assessed as the kinetics of the protein in the Golgi area. The kinetics was defined as a change in the ratio of the fluorescent intensities of VSV-G(ts045)–GFP in the Golgi area to those in the whole cell over time. Post-Golgi trafficking of VSV-G(ts045) was significantly delayed in infected N2aC24L1-3 and N2aC24Chm cells, compared with that in uninfected N2aC24 cells. Blue and greenP-values indicate significances of infected cells against those of uninfected or cured cells, respectively. No significant difference in the VSV-G(ts045)–GFP trafficking was observed between uninfected N2aC24 and cured N2aC24L1-3 or cured N2aC24Chm cells. Data were analysed using the Student’st-test. Figure 1: Post-Golgi vesicular trafficking is delayed in 22L prion-infected N2aC24L1-3 and Chandler prion-infected N2aC24Chm cells. ( a ) Upper panels: WB of uninfected N2aC24, infected N2aC24L1-3 and cured N2aC24L1-3 cells with 6D11 anti-PrP Ab. Lower panels: WB of uninfected N2aC24, infected N2aC24Chm and cured N2aC24Chm cells with 6D11 anti-PrP Ab. PrP Sc was detected in infected N2aC24L1-3 or N2aC24Chm cells, but not in uninfected N2aC24, cured N2aC24L1-3, and cured N2aC24Chm cells. Each cell lysate was treated without (−) or with (+) PK. β-Actin is an internal control. ( b ) Transport assay of VSV-G(ts045)–GFP in uninfected N2aC24, infected N2aC24L1-3 and cured N2aC24L1-3 cells. ( c ) Transport assay of VSV-G(ts045)–GFP in uninfected N2aC24, infected N2aC24Chm and cured N2aC24Chm cells. Cells were transfected with the vector encoding VSV-G(ts045)–GFP and incubated at the non-permissive temperature at 39.5 °C. Fluorescent intensities for VSV-G(ts045)–GFP at the Golgi region against those in the whole cell were determined in the randomly selected transfected cells ( n =14–16) at various times, after the cells were transferred to the permissive temperature of 32 °C. Trafficking of VSV-G(ts045)–GFP in the cells was assessed as the kinetics of the protein in the Golgi area. The kinetics was defined as a change in the ratio of the fluorescent intensities of VSV-G(ts045)–GFP in the Golgi area to those in the whole cell over time. Post-Golgi trafficking of VSV-G(ts045) was significantly delayed in infected N2aC24L1-3 and N2aC24Chm cells, compared with that in uninfected N2aC24 cells. Blue and green P -values indicate significances of infected cells against those of uninfected or cured cells, respectively. No significant difference in the VSV-G(ts045)–GFP trafficking was observed between uninfected N2aC24 and cured N2aC24L1-3 or cured N2aC24Chm cells. Data were analysed using the Student’s t -test. Full size image To assess prion infection on the transport of VSV-G(ts045)–GFP, uninfected N2aC24, infected N2aC24L1-3 and cured N2aC24L1-3 cells were transiently transfected with the VSV-G(ts045)–GFP expression vector at 39.5 °C and, 16 h after transfection, cultured at 32 °C with the protein synthesis inhibitor cycloheximide allowing monitoring of the already synthesized VSV-G(ts045)–GFP alone. The cells were fixed at various time points immediately after the culture was started at 32 °C and stained with Abs against GFP and the Golgi marker GM130 by immunohistochemistry (IHC). The fluorescent intensities of VSV-G(ts045)–GFP in the whole cell and the GM130-positive area were measured. About 10% of total VSV-G(ts045)–GFP was detected at the GM130-positive area in these cells at 0 min at 32 °C ( Fig. 1b ; Supplementary Fig. S1 ). This might be because a small portion of VSV-G(ts045)–GFP in the ER overlaps with the Golgi apparatus or is resistant to the non-permissive temperature, exiting from the ER to the Golgi apparatus, or both. As soon as the culture was started at 32 °C, VSV-G(ts045)–GFP began to accumulate in the Golgi apparatus with similar kinetics in the cells, reaching maximum at 30 min ( Fig. 1b ; Supplementary Fig. S1 ), indicating that vesicular trafficking of VSV-G(ts045)–GFP from the ER to the Golgi apparatus was not affected by prion infection. However, after 30 min at 32 °C, infected cells showed significantly delayed decreased VSV-G(ts045)–GFP fluorescent intensities in the Golgi apparatus, compared with uninfected cells ( Fig. 1b ; Supplementary Fig. S1 ). This delayed decrease was rescued in cured cells ( Fig. 1b ; Supplementary Fig. S1 ). Similar delayed decrease in the fluorescent intensities of VSV-G(ts045)–GFP in the Golgi apparatus was observed in N2aC24Chm cells, N2aC24 cells persistently infected with Chandler prions ( Fig. 1a ). This delayed decrease was also recovered in cured N2aC24Chm cells ( Fig. 1a ). These results indicate that post-Golgi trafficking of VSV-G(ts045)–GFP was delayed in infected cells. We further investigated the levels of VSV-G(ts045)–GFP transported to the cell surface using fluorescence-activated cell sorter (FACS) analysis. The transfected cells were cultured for 120 min at 32 °C with cycloheximide and then immediately subjected to FACS analysis. The cells expressing VSV-G(ts045)–GFP were detected by the GFP fluorescence, and VSV-G(ts045)–GFP transported to the cell surface were detected with anti-VSV-G Ab and DyLight 649-conjugated Ab ( Supplementary Fig. S2a,b ). The fluorescent signal corresponding to the surface VSV-G(ts045)–GFP was significantly lower in infected cells than in uninfected or cured cells ( Supplementary Fig. S2a,b ), indicating that VSV-G(ts045)–GFP transport was delayed to the cell surface in infected cells. Impaired post-Golgi transport of PrP C in infected cells We investigated whether the post-Golgi trafficking of PrP C to the cell surface might be impaired in infected cells. We first semi-quantified PrP C expressed on the surface of uninfected N2aC24, infected N2aC24L1-3 and cured N2aC24L1-3 cells using biotin labelling of cell surface proteins. The labelled proteins were purified by avidin beads and subjected to WB with 6D11 anti-PrP Ab against an epitope within residues 93–109. Total PrP was increased because of the accumulation of PrP Sc in infected cells ( Fig. 2a ). However, the biotinylated PrP levels were lower in infected cells, compared with uninfected cells ( Fig. 2a ). Reduced levels were recovered in cured cells ( Fig. 2a ). Less than 1% of the biotinylated PrP from infected cells were PK resistant ( Fig. 2c ), indicating that most of the biotinylated PrP are PrP C . These results indicate that surface PrP C is reduced in prion-infected cells. 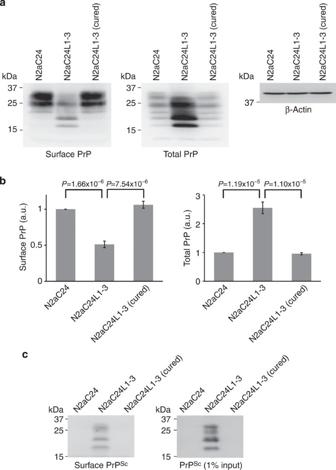Figure 2: Cell surface expression of PrPCis decreased in infected cells. (a) WB with 6D11 anti-PrP Ab of biotin-labelled surface PrP and total PrP in uninfected N2aC24, infected N2aC24L1-3 and cured N2aC24L1-3 cells. Surface expression of PrP was reduced in infected N2aC24L1-3 cells, compared with that in uninfected N2aC24 and cured N2aC24L1-3 cells (left panel). Total PrP were increased in infected N2aC24L1-3 cells, due to accumulation of PrPSc(middle panel). β-Actin is an internal control (right panel). (b) Signal densities for PrP in each lane against those for β-actin were statistically analysed from three independent experiments using the Student’st-test. Vertical axes are indicated as an arbitrary unit (a.u.). Error bars, s.d. (c) WB of the purified and unpurified biotinylated PrP after PK treatment. Less than 1% of the biotinylated PrP from infected N2aC24L1-3 cells were PK resistant, indicating most biotinylated PrP are PrPC. Figure 2: Cell surface expression of PrP C is decreased in infected cells. ( a ) WB with 6D11 anti-PrP Ab of biotin-labelled surface PrP and total PrP in uninfected N2aC24, infected N2aC24L1-3 and cured N2aC24L1-3 cells. Surface expression of PrP was reduced in infected N2aC24L1-3 cells, compared with that in uninfected N2aC24 and cured N2aC24L1-3 cells (left panel). Total PrP were increased in infected N2aC24L1-3 cells, due to accumulation of PrP Sc (middle panel). β-Actin is an internal control (right panel). ( b ) Signal densities for PrP in each lane against those for β-actin were statistically analysed from three independent experiments using the Student’s t -test. Vertical axes are indicated as an arbitrary unit (a.u.). Error bars, s.d. ( c ) WB of the purified and unpurified biotinylated PrP after PK treatment. Less than 1% of the biotinylated PrP from infected N2aC24L1-3 cells were PK resistant, indicating most biotinylated PrP are PrP C . Full size image We performed IHC of these cells using SAF83 anti-PrP Ab against an epitope within residues 126–164 under standard conditions of fixation and permeabilization, in which most PrP Sc escapes labelling by the Ab. Hence, PrP C is preferentially visualized. Consistent with PrP C being a membrane glycoprotein, uninfected cells exhibited strong cell surface signals ( Fig. 3a ). However, in infected cells, a region near the nucleus, detected by anti-lamin A Ab, was aberrantly stained ( Fig. 3a ). The cell surface signals were still detectable but decreased in infected cells ( Fig. 3a ). The aberrant staining near the nucleus was absent in cured cells ( Fig. 3a ). We also costained infected cells with Abs against various organelle markers. Most of the SAF83-positive signals were costained with the Golgi markers, more strongly with the trans -Golgi network marker TGN38 than with the cis -Golgi marker giantin ( Fig. 3b ). Not all of the SAF83-positive signals were precisely costained with the trans -Golgi markers. The trans -Golgi network consists of distinct subcompartments [24] . Therefore, PrP C might be preferentially accumulated in a specific trans -Golgi network subcompartment(s). A small proportion of the signals were stained with the recycling endosome markers, Rab11 and transferrin receptor (TfR), and the early endosome marker, EEA1 ( Fig. 3b ). These results indicate that, in prion-infected cells, PrP C is aberrantly present in the Golgi apparatus and only a small proportion of it can enter into the post-Golgi vesicular transport pathway. 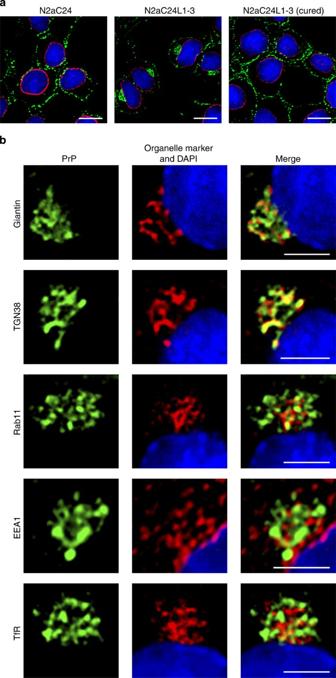Figure 3: Aberrant accumulation of PrPCin the Golgi apparatus in infected cells. (a) Uninfected N2aC24, infected N2aC24L1-3 and cured N2aC24L1-3 cells were immunohistochemically stained with SAF83 anti-PrP Ab (green). Most signals were observed on the cell surface in uninfected N2aC24 and cured N2aC24L1-3 cells. In contrast, the surface signal was reduced and a region near the nucleus became stained in infected N2aC24L1-3 cells. The nuclear envelope was stained with anti-lamin A Ab (red). The nucleus was stained with DAPI (blue). (b) Costaining of PrPCin infected N2aC24L1-3 cells with thecis-Golgi marker giantin, thetrans-Golgi network marker TGN38, the recycling endosome markers Rab11 and TfR, and the early endosome marker EEA1. The PrP signal in the region near the nucleus was preferentially costained with the Golgi markers, particularly with thetrans-Golgi network marker, TGN38, in infected N2aC24L1-3 cells. Green fluorescence, PrP; blue fluorescence, nucleus; red fluorescence, the organelle markers; yellow fluorescence, combined signals. Scale bars 5 μm. Figure 3: Aberrant accumulation of PrP C in the Golgi apparatus in infected cells. ( a ) Uninfected N2aC24, infected N2aC24L1-3 and cured N2aC24L1-3 cells were immunohistochemically stained with SAF83 anti-PrP Ab (green). Most signals were observed on the cell surface in uninfected N2aC24 and cured N2aC24L1-3 cells. In contrast, the surface signal was reduced and a region near the nucleus became stained in infected N2aC24L1-3 cells. The nuclear envelope was stained with anti-lamin A Ab (red). The nucleus was stained with DAPI (blue). ( b ) Costaining of PrP C in infected N2aC24L1-3 cells with the cis -Golgi marker giantin, the trans -Golgi network marker TGN38, the recycling endosome markers Rab11 and TfR, and the early endosome marker EEA1. The PrP signal in the region near the nucleus was preferentially costained with the Golgi markers, particularly with the trans -Golgi network marker, TGN38, in infected N2aC24L1-3 cells. Green fluorescence, PrP; blue fluorescence, nucleus; red fluorescence, the organelle markers; yellow fluorescence, combined signals. Scale bars 5 μm. Full size image We confirmed if PrP molecules aberrantly accumulated in the Golgi apparatus in prion-infected cells are PrP C rather than PrP Sc , by transfecting the expression vector encoding hamster or human PrP C into uninfected N2aC24, infected N2aC24L1-3 and cured N2aC24L1-3 cells. Human and hamster PrP C s do not undergo structural conversion into PrP Sc in cells infected with mouse-derived prions. Indeed, no PK-resistant human and hamster PrPs were detected on WB of the transfected N2aC24L1-3 cells using 3F4 anti-PrP Ab, which specifically detects hamster and human PrPs ( Supplementary Fig. S3a,b ). However, aberrant staining of hamster and human PrP C near the nucleus was observed in infected cells, but not in uninfected or cured cells ( Supplementary Fig. S3c ). Most PrP Sc is in recycling endosome in infected cells To investigate the mechanism of prion infection-induced impairment of post-Golgi vesicular trafficking, we investigated subcellular localization of PrP Sc in infected cells by performing PrP Sc -specific IHC with anti-PrP monoclonal Ab mAb132. The mAb132 was demonstrated to recognize the residues 119–127 of mouse PrP, and specifically visualize PrP Sc under partially denatured conditions [25] . No signals were detected in uninfected N2aC24 and cured N2aC24L1-3 cells ( Fig. 4a ). In contrast, strong signals were observed near the nucleus in infected N2aC24L1-3 and N2aC24Chm cells ( Fig. 4a ). The signals were not costained with the nuclear membrane marker lamin ( Fig. 4a ). We also costained PrP Sc with other organelle markers. Only a small proportion of PrP Sc were costained with giantin and TGN38 ( Fig. 4b ). In contrast, most PrP Sc were costained with Rab11, TfR, EEA1 and the late endosome marker Rab9 ( Fig. 4b ). The strongest staining of PrP Sc was observed in the TfR-positive recycling endosome ( Fig. 4b ). We found similar staining of PrP Sc in N2aC24Chm cells ( Fig. 4b ). These results indicate that in infected cells, PrP Sc is mainly accumulated throughout endosomal compartments and particularly abundantly in the TfR-positive recycling endosome, but little in the Golgi apparatus. Recycling endosome might consist of distinct compartments. Thus, PrP Sc could be preferentially accumulated in a distinct compartment(s), such as the TfR-positive recycling endosome compartment. 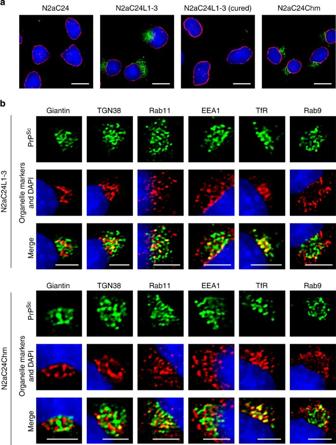Figure 4: Subcellular localization of PrPScin infected cells. (a) PrPSc(green) was detected using mAb132 in infected N2aC24L1-3 and N2aC24Chm cells under partially denatured conditions. No signals were detected in uninfected N2aC24 and cured N2aC24L1-3 cells. In contrast, strong signals corresponding to PrPScwere detected in infected N2aC24L1-3 and N2aC24Chm cells. The nuclear envelope was stained with anti-lamin A Ab (red). The nucleus was stained with DAPI (blue). (b) PrPScwas costained with thecis-Golgi marker giantin, thetrans-Golgi network marker TGN38, the recycling endosome markers Rab11 and TfR, and the early endosome marker EEA1, and the late endosome maker Rab9 in infected N2aC24L1-3 and N2aC24Chm cells. PrPScis mainly accumulated throughout endosomal compartments, particularly abundantly in the TfR-positive recycling endosome, but little in the Golgi apparatus. Green fluorescence, PrP; blue fluorescence, nucleus; red fluorescence, the organelle markers; yellow fluorescence, combined signals. Scale bars 5 μm. Figure 4: Subcellular localization of PrP Sc in infected cells. ( a ) PrP Sc (green) was detected using mAb132 in infected N2aC24L1-3 and N2aC24Chm cells under partially denatured conditions. No signals were detected in uninfected N2aC24 and cured N2aC24L1-3 cells. In contrast, strong signals corresponding to PrP Sc were detected in infected N2aC24L1-3 and N2aC24Chm cells. The nuclear envelope was stained with anti-lamin A Ab (red). The nucleus was stained with DAPI (blue). ( b ) PrP Sc was costained with the cis -Golgi marker giantin, the trans -Golgi network marker TGN38, the recycling endosome markers Rab11 and TfR, and the early endosome marker EEA1, and the late endosome maker Rab9 in infected N2aC24L1-3 and N2aC24Chm cells. PrP Sc is mainly accumulated throughout endosomal compartments, particularly abundantly in the TfR-positive recycling endosome, but little in the Golgi apparatus. Green fluorescence, PrP; blue fluorescence, nucleus; red fluorescence, the organelle markers; yellow fluorescence, combined signals. Scale bars 5 μm. Full size image Surface attractin is reduced in infected cells We asked whether impaired post-Golgi vesicle transport could be relevant to the pathogenesis of prion diseases. Loss of attractin function was shown to cause prion disease-like spongiform changes in the brains of animals [22] . Therefore, we semi-quantified cell surface attractin in uninfected N2aC24, infected N2aC24L1-3 and cured N2aC24L1-3 cells, using biotin labelling of cell surface proteins. The surface expression of attractin was reduced in infected cells, compared with uninfected cells ( Fig. 5a ). The reduced surface expression of attractin was recovered in cured cells ( Fig. 5a ). Total attractin was the same for all three groups of cells ( Fig. 5a ), indicating that the reduced surface expression of attractin in infected cells is not due to downregulation of attractin expression. These results indicate that prion infection could reduce the cell surface expression of attractin. 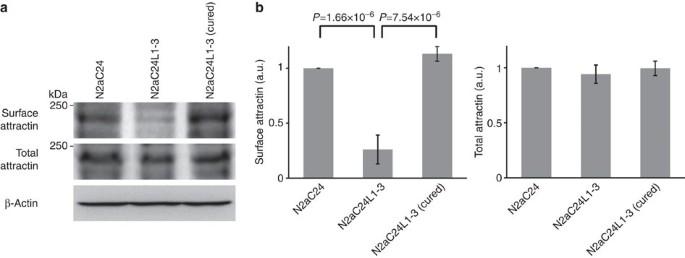Figure 5: Decreased surface attractin in infected cells. (a) WB of biotin-labelled surface attractin and total attractin in uninfected N2aC24, infected N2aC24L1-3, and cured N2aC24L1-3 cells. Surface expression of attractin was reduced in infected N2aC24L1-3 cells, compared with uninfected N2aC24 and cured N2aC24L1-3 cells. No reduction of total attractin was detected in infected N2aC24L1-3 cells. β-Actin is an internal control. (b) Signal densities for attractin in each lane against those for β-actin were statistically analysed from three independent experiments using the Student’st-test. Error bars, s.d. Figure 5: Decreased surface attractin in infected cells. ( a ) WB of biotin-labelled surface attractin and total attractin in uninfected N2aC24, infected N2aC24L1-3, and cured N2aC24L1-3 cells. Surface expression of attractin was reduced in infected N2aC24L1-3 cells, compared with uninfected N2aC24 and cured N2aC24L1-3 cells. No reduction of total attractin was detected in infected N2aC24L1-3 cells. β-Actin is an internal control. ( b ) Signal densities for attractin in each lane against those for β-actin were statistically analysed from three independent experiments using the Student’s t -test. Error bars, s.d. Full size image Surface IR and insulin signal are reduced in infected cells To further assess the relevance of the impaired post-Golgi trafficking to the pathogenesis of prion diseases, we asked whether the reduced surface expression of membrane proteins could disturb downstream signalling in infected cells. The IR-mediated signal is neuroprotective and its impaired signal may be involved in the pathogenesis of neurodegenerative disorders [14] , [15] , [16] , [17] . We thus semi-quantified the cell surface expression of the α-subunit of insulin receptor (IRα) in uninfected N2aC24, infected N2aC24L1-3 and cured N2aC24L1-3 cells using biotin labelling of cell surface proteins. The surface expression of IRα was reduced in infected cells, compared with uninfected cells ( Fig. 6a ). The reduced expression of the molecule was recovered in cured cells ( Fig. 6a ). IHC revealed that the molecule was aberrantly accumulated in the Golgi apparatus, which was stained with anti-GM130 Ab, in infected cells but not in uninfected or cured cells ( Fig. 6c ). These results indicate that prion infection could reduce the cell surface expression of IRα by impairing post-Golgi trafficking. 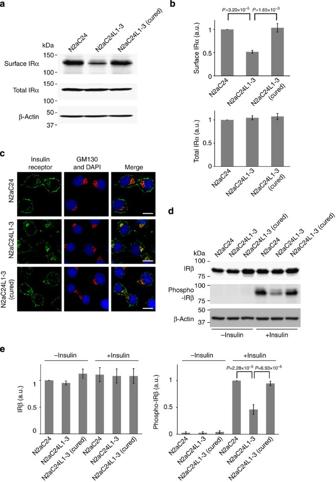Figure 6: Suppressed insulin signal in infected cells. (a) WB of biotin-labelled surface IRα and total IRα in uninfected N2aC24, infected N2aC24L1-3 and cured N2aC24L1-3 cells. Surface expression of IRα was reduced in infected N2aC24L1-3 cells, compared with uninfected N2aC24 and cured N2aC24L1-3 cells. No reduction of total IRα was detected in infected N2aC24L1-3 cells. β-Actin is an internal control. (b) Signal densities for the subunit in each lane against those for β-actin were statistically analysed from three independent experiments using the Student’st-test. Error bars, s.d. (c) IHC of IRα (green) and the Golgi marker GM130 (red) in uninfected N2aC24, infected N2aC24L1-3 and cured N2aC24L1-3 cells. IRα was costained with the Golgi marker GM130 in infected N2aC24L1-3 cells, but not in uninfected N2aC24, and cured N2aC24L1-3 cells. Blue fluorescence, nucleus; yellow fluorescence, combined signals. Scale bars 10 μm. (d) WB of total IRβ and phosphorylated β-subunit (phospho-IRβ) in uninfected N2aC24, infected N2aC24L1-3 and cured N2aC24L1-3 cells after insulin stimulation. Total amounts of IRβ were similar among these different cell types. However, insulin-stimulated autophosphorylation of IRβ was suppressed in infected N2aC24L1-3 cells. β-Actin is an internal control. (e) Signal densities for IRβ in each lane against those for β-actin were statistically analysed from three independent experiments using the Student’st-test. Error bars, s.d. Figure 6: Suppressed insulin signal in infected cells. ( a ) WB of biotin-labelled surface IRα and total IRα in uninfected N2aC24, infected N2aC24L1-3 and cured N2aC24L1-3 cells. Surface expression of IRα was reduced in infected N2aC24L1-3 cells, compared with uninfected N2aC24 and cured N2aC24L1-3 cells. No reduction of total IRα was detected in infected N2aC24L1-3 cells. β-Actin is an internal control. ( b ) Signal densities for the subunit in each lane against those for β-actin were statistically analysed from three independent experiments using the Student’s t -test. Error bars, s.d. ( c ) IHC of IRα (green) and the Golgi marker GM130 (red) in uninfected N2aC24, infected N2aC24L1-3 and cured N2aC24L1-3 cells. IRα was costained with the Golgi marker GM130 in infected N2aC24L1-3 cells, but not in uninfected N2aC24, and cured N2aC24L1-3 cells. Blue fluorescence, nucleus; yellow fluorescence, combined signals. Scale bars 10 μm. ( d ) WB of total IRβ and phosphorylated β-subunit (phospho-IRβ) in uninfected N2aC24, infected N2aC24L1-3 and cured N2aC24L1-3 cells after insulin stimulation. Total amounts of IRβ were similar among these different cell types. However, insulin-stimulated autophosphorylation of IRβ was suppressed in infected N2aC24L1-3 cells. β-Actin is an internal control. ( e ) Signal densities for IRβ in each lane against those for β-actin were statistically analysed from three independent experiments using the Student’s t -test. Error bars, s.d. Full size image We then investigated whether reduced surface expression of IRα could affect the downstream signal in infected cells. Upon binding of insulin to the receptor, the β-subunit of the receptor (IRβ) undergoes autophosphorylation of tyrosine residues at 1,150 and 1,151 in the intracellular domain. Therefore, we assessed the phosphorylation level of IRβ in infected cells using WB with a mAb able to recognize the epitope including these phosphorylated tyrosine residues. Increased levels of the phosphorylated IRβ were observed in these cells after stimulation with insulin ( Fig. 6d ). However, the phosphorylation level was much lower in infected cells than in uninfected or cured cells ( Fig. 6d ). These results indicate that reduced surface expression of the IR could weaken the insulin signal in infected cells. Surface PrP C , IR and attractin are reduced in ScN2a cells Infected N2aC24L1-3 cells overexpress exogenously transfected mouse PrP C , raising the possibility that impaired post-Golgi trafficking, eventually reducing surface expression of membrane proteins, might be due to the overexpression of PrP C but not to prion infection. ScN2a cell line is a widely used prion-infected N2a cell line that expresses endogenous PrP C alone ( Supplementary Fig. S4a ). To rule out the possibility, we semi-quantified the cell surface expression of PrP C , the IRα and attractin in uninfected N2a and ScN2a cells using biotin labelling of cell surface proteins. Surface expression of all of the molecules was significantly reduced in ScN2a cells, compared with those in uninfected N2a cells ( Supplementary Fig. S4b–g ). These results clearly indicate that the impaired post-Golgi trafficking detected in infected N2aC24L1-3 cells is due to prion infection not due to the overexpression of PrP C . Prions reduce surface PrP C and IR in mouse brains We finally asked whether the post-Golgi trafficking of membrane proteins is impaired in prion-infected brains. We thus investigated the surface expression levels of PrP C and IRα in the brains of mice infected with RML and 22L prions. Coronally sliced fresh brains removed from terminally ill mice were subjected to surface biotin labelling ( Fig. 7a ). Total IRα was the same for both uninfected and infected brains, and total PrP was increased in infected brains due to accumulation of PrP Sc ( Fig. 7b–d ). However, biotinylated IRα and PrP C were significantly lower in infected brains than in uninfected brains ( Fig. 7b–d ), indicating that surface expression of PrP C and IRα was decreased in infected brains. We also investigated another GPI-anchored membrane molecule, Thy-1 (ref. 26 ), and two multipass transmembrane molecules, the glutamate receptor subunits GluR3 and NR1 (ref. 27 ), for their surface levels in infected brains. Surface expression of Thy-1 was significantly reduced in infected brains compared with uninfected brains ( Supplementary Fig. S5a,b ). In contrast, GluR3 and NR1 were similarly expressed on the cell surface of both uninfected and infected brains ( Supplementary Fig. S5a,c,d ). These results indicate that prion infection could impair the post-Golgi trafficking of some but not all membrane proteins. 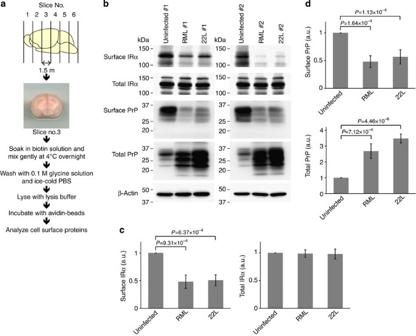Figure 7: Surface PrPCand the insulin receptor is reduced in prion-infected mouse brains. (a) The simplified protocol for biotin labelling of surface proteins in mouse brains. Brain tissues were removed from terminally ill mice-infected RML and 22L scrapie prions and from PBS-inoculated age-matched ICR mice at the same time, immediately sectioned into 1.5-mm-thick sections and then the surface proteins were biotinylated. The biotinylated proteins were analysed using WB. (b) WB of biotin-labelled surface IRα and total IRα, and biotin-labelled surface PrPCand total PrP in the brains of mice infected with RML and 22L prions. The results were shown for two independent mouse brains from each group. PrP was detected with 6D11 anti-PrP Ab. Uninfected controls were PBS-inoculated age-matched mice. Total IRα was the same in uninfected and infected brains, and total PrP was increased in infected brains due to accumulation of PrPSc. However, biotinylated IRα and PrPCwere significantly lower in infected brains than in uninfected brains. β-Actin is an internal control. Signal densities for IRα (c) and PrP (d) in each lane against those for β-actin were statistically analysed for four independent mouse brains from each group using the Student’st-test. Error bars, s.d. Figure 7: Surface PrP C and the insulin receptor is reduced in prion-infected mouse brains. ( a ) The simplified protocol for biotin labelling of surface proteins in mouse brains. Brain tissues were removed from terminally ill mice-infected RML and 22L scrapie prions and from PBS-inoculated age-matched ICR mice at the same time, immediately sectioned into 1.5-mm-thick sections and then the surface proteins were biotinylated. The biotinylated proteins were analysed using WB. ( b ) WB of biotin-labelled surface IRα and total IRα, and biotin-labelled surface PrP C and total PrP in the brains of mice infected with RML and 22L prions. The results were shown for two independent mouse brains from each group. PrP was detected with 6D11 anti-PrP Ab. Uninfected controls were PBS-inoculated age-matched mice. Total IRα was the same in uninfected and infected brains, and total PrP was increased in infected brains due to accumulation of PrP Sc . However, biotinylated IRα and PrP C were significantly lower in infected brains than in uninfected brains. β-Actin is an internal control. Signal densities for IRα ( c ) and PrP ( d ) in each lane against those for β-actin were statistically analysed for four independent mouse brains from each group using the Student’s t -test. Error bars, s.d. Full size image We then addressed whether or not post-Golgi trafficking could be affected in infected brains of symptom-free mice, by similarly assessing the surface levels of IRα and PrP C in infected brains removed at 2, 62–68 and 80–87 days post inoculation (dpi) with RML prions. The inoculated mice developed the disease around at 112 dpi. PrP Sc was detected at 68 dpi, with increased amounts at 87 dpi, reaching its maximal level at the terminal stage ( Supplementary Fig. S6a ). No difference was observed in the levels of surface IRα and PrP C in uninfected and infected brains at 2 dpi ( Supplementary Fig. S6b–d ). However, at 80–87 dpi, the surface IRα and PrP C were significantly lower in infected brains than in uninfected brains ( Supplementary Fig. S6b–d ). They also appeared lower in infected brains at 62–68 dpi ( Supplementary Fig. S6b–d ). These results indicate that post-Golgi trafficking is impaired in infected brains of mice well before the onset of clinical symptoms. In the present study, we showed that post-Golgi vesicular trafficking was delayed in N2a cells persistently infected with 22L or Chandler prions, N2aC24L1-3 and N2aC24Chm cells. This delayed trafficking was successfully rescued in cured cells, clearly indicating that it is due to the prion infection. Impairment of the vesicle trafficking could have adverse effects because membrane proteins important for normal cellular functions, such as adhesion molecules, ion channels, or receptors, may not be correctly delivered to the plasma membrane. Indeed, we found that membrane proteins examined, including PrP C , IRα and attractin, had reduced surface expression in infected N2aC24L1-3 cells. We also showed that surface expression of PrP C , IRα and attractin were reduced in prion-infected ScN2a cells. Furthermore, surface expression of PrP C , IRα and Thy-1 were reduced in the brains of mice infected with RML and 22L prions. However, the surface expression of GluR3 and NR1 was not affected. PrP C and Thy-1 are GPI-anchored molecules, IR and attractin are single-pass transmembrane molecules, and GluR3 and NR1 are multipass transmembrane molecules. These results suggest that prion infection might impair the post-Golgi trafficking of certain types of membrane proteins, causing neuronal dysfunctions associated with prion disease. Mice tg for the GPI-anchored membrane protein PrP-EGFP, a fusion protein of PrP with EGFP, were reported to exhibit aberrant accumulation of PrP-EGFP in the Golgi apparatus in neurons after infection with RML prions [9] . PrP-EGFP itself did not undergo conformational conversion and therefore failed to support prion propagation in mice [9] . These results reinforce our conclusion that prion infection could disturb the post-Golgi trafficking of membrane proteins to the cell surface, inducing aberrant accumulation of them in the Golgi apparatus. Interestingly, accumulation of PrP-EGFP in the Golgi apparatus in the mice was observed from the early stages after infection [9] , suggesting that impairment of post-Golgi trafficking might be an early pathogenic event in prion disease. Consistent with this idea, we showed that the surface expression of IRα and PrP C was reduced in infected mouse brains well before the onset of clinical symptoms. It remains controversial whether loss-of-function of PrP C is involved in the pathogenesis of prion disease. We previously found demyelination in the spinal cord and peripheral nerves of Prnp 0/0 mice regardless of the ectopic expression of a PrP-like molecule, Dpl [28] . Other investigators reported that Prnp 0/0 mice displayed altered sleep patterns and circadian rhythms, and impaired long-term potentiation thought to be an electrophysiological mechanism underlying defective memory and learning [29] , [30] . These abnormal phenotypes in Prnp 0/0 mice are often reported in patients affected with prion diseases. However, Prnp 0/0 mice developed neither spongiform neurodegeneration nor neuronal cell loss [31] . Therefore, loss-of-function of PrP C might be responsible for only some aspects of the pathogenic features in prion diseases, such as those observed in Prnp 0/0 mice, but not for spongiform degeneration and neuronal cell death. PrP C is synthesized in the ER, transits the Golgi apparatus and is delivered to the cell surface, where it resides in lipid rafts, suggesting that PrP C might play roles as a membrane receptor and adhesion molecule. We showed that the surface expression of PrP C was reduced in infected N2aC24L1-3 and ScN2a cells and in infected mouse brains. It is thus possible that the reduced surface expression of PrP C might lead to its functional deficiency in prion-infected cells, thereby causing some aspects of the pathogenic features in prion diseases, such as those observed in Prnp 0/0 mice. Spongiform neurodegeneration is a pathological hallmark of prion diseases. Loss-of-function for attractin, a large transmembrane protein that is conserved among animals, is known to cause prion disease-like spongiform neurodegeneration [22] . Similar spongiform neurodegeneration is reported in mice lacking functional mahogunin, a cytosolic E3 ubiquitin ligase, suggesting that mahogunin is a downstream molecule of attractin [32] . Mahogunin has already been shown to be functionally impaired by binding to Ctm PrP or cytosolic PrP, suggesting that functional deficiency of mahogunin might be involved in spongiform formation in prion disease [33] . Here, we showed that cell surface expression of attractin was reduced in prion-infected cells due to impairment of post-Golgi trafficking. These results suggest that impairment of post-Golgi trafficking might be involved in spongiform degeneration in prion diseases by causing functional impairment of the attractin/mahogunin pathway in prion-infected neurons. We also found that the cell surface expression of the IRα was reduced in infected N2aC24L1-3 and ScN2a cells and in infected mouse brains, and that autophosphorylation of the IRβ was suppressed in infected N2aC24L1-3 cells after stimulation with insulin. Reduced insulin signalling is suggested to be involved in the pathogenesis of neurodegenerative disorders, such as Alzheimer’s disease, by reducing its neuroprotective function and dysregulating synaptic plasticity and memory formation [14] , [15] , [16] , [17] , [18] , [19] , [20] , [21] . These results suggest that dysfunction of the insulin signal that is evoked by reduction of the cell surface expression of the IRα due to the prion infection-mediated impairment of post-Golgi vesicular trafficking might be involved in the pathogenesis of prion diseases. We showed that PrP C and IR were aberrantly accumulated in the Golgi apparatus. It has been reported that abnormal accumulation of membrane or secretory proteins in the Golgi apparatus could induce ER stress [34] . Elevation of ER stress was reported in prion-infected cells and brains [35] , [36] , suggesting that ER stress-mediated apoptosis might be responsible for neuronal cell death in prion diseases. Therefore, aberrantly accumulated membrane proteins, such as PrP C and the IR, caused by the impaired post-Golgi vesicular trafficking might induce ER stress and eventually apoptosis in infected cells. In contrast to the aberrant accumulation of PrP C in the Golgi apparatus, only a very small proportion of PrP Sc was detected in the Golgi apparatus of infected cells. This is consistent with previous reports by other investigators using other prion-infected cells [8] , [25] . Instead, most PrP Sc was observed throughout endosomal compartments, being particularly abundant in recycling endosome in infected cells. Similar subcellular distribution of PrP Sc was shown by others [25] . Accumulation of PrP Sc in recycling endosome was also shown in neurons of RML prion-infected mice [37] . Membrane or secretory proteins synthesized in the ER were first transported to the Golgi apparatus and then to the plasma membrane either directly or via recycling endosome [38] , [39] . Therefore, abnormal accumulation of PrP Sc in recycling endosome could disturb vesicle transport from the Golgi apparatus to the recycling endosome and then to the plasma membrane ( Fig. 8 ). Some proteins in recycling endosomes are retrograded to the Golgi apparatus [40] . A small proportion of PrP Sc also might be transported from the recycling endosome to the Golgi apparatus using the same pathway. Massignan et al . [41] reported that the PrP mutant D178N/Met-129 linked to fatal familial insomnia was abnormally accumulated in the ER and Golgi apparatus of transfected N2a cells and impaired post-Golgi vesicular trafficking by inducing the Rab GDP dissociation inhibitor α expression and, in contrast, by reducing Rab11. These results suggest that impairment of the post-Golgi trafficking also could be involved in the pathogenesis of hereditary prion diseases. However, the accumulation site for PrP Sc and the mutant PrP was different, suggesting different mechanisms underlying the disturbed post-Golgi vesicular trafficking in acquired and hereditary prion diseases. 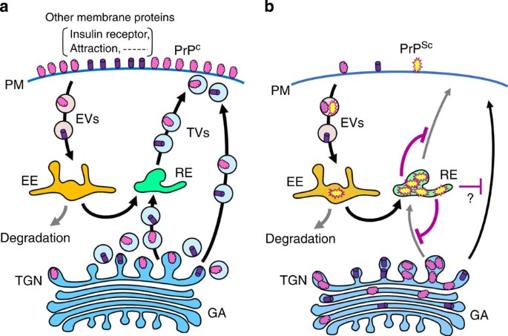Figure 8: A hypothetical pathogenic mechanism of prion disease. (a) In uninfected neurons, membrane proteins synthesized in the ER are normally delivered to the plasma membrane (PM) via the Golgi apparatus (GA) using a vesicular trafficking system. (b) In infected neurons, PrPScpreferentially accumulated at recycling endosomes (REs) impairs post-Golgi vesicular trafficking of membrane proteins, such as PrPC, IR and attractin, to the PM, causing functional deficiency of each molecule and finally inducing neuronal dysfunctions involved in the pathogenesis of prion diseases. EE, early endosome; EVs, endocytic vesicles; TGN, the trans-Golgi network; TVs, transport vesicles. Figure 8: A hypothetical pathogenic mechanism of prion disease. ( a ) In uninfected neurons, membrane proteins synthesized in the ER are normally delivered to the plasma membrane (PM) via the Golgi apparatus (GA) using a vesicular trafficking system. ( b ) In infected neurons, PrP Sc preferentially accumulated at recycling endosomes (REs) impairs post-Golgi vesicular trafficking of membrane proteins, such as PrP C , IR and attractin, to the PM, causing functional deficiency of each molecule and finally inducing neuronal dysfunctions involved in the pathogenesis of prion diseases. EE, early endosome; EVs, endocytic vesicles; TGN, the trans-Golgi network; TVs, transport vesicles. Full size image In short, we showed here that prion infection could disturb the post-Golgi vesicular trafficking of some but not all membrane proteins to the cell surface, and suggested that the disturbed post-Golgi vesicular trafficking could eventually cause neuronal dysfunctions associated with the pathogenesis of prion disease. For further understanding of the pathogenesis of prion diseases and development of treatments for prion diseases, it might be worth investigating the molecular mechanism underlying the impaired post-Golgi vesicular trafficking in prion-infected cells. Ethics statement The Ethics Committee of Animal Care and Experimentation of The University of Tokushima approved this study (approval number 11002). Animals were cared for in accordance with The Guiding Principle for Animal Care and Experimentation of The University of Tokushima and Japanese Law for Animal Welfare and Care. Abs and reagents The Abs used in this study are: rabbit polyclonal anti-giantin (1:1,000) (Covance, Emeryville, CA), rabbit polyclonal anti-TGN38 (1:500) (Novus Biologicals, Littleton, CO), anti-EEA1 (1:500) (Novus Biologicals), rabbit polyclonal anti-Rab11 (1:500) (Cell Signaling, Danvers, MA), rabbit monoclonal anti-Rab9 (D52G8) (1:500) (Cell signaling), rabbit monoclonal anti-IRβ (4B8) (1:1,000) (Cell Signaling), rabbit monoclonal anti-phospho-IR (19H7) (Tyr1150/1151) (1:500) (Cell Signaling), rabbit polyclonal anti-TfR (1:500) (Abcam, Cambridge, UK), rabbit polyclonal anti-IRα (1:200 for IHC, 1:500 for WB) (Santa Cruz Biotechnology Inc., Santa Cruz, CA), rabbit polyclonal anti-attractin (1:200) (Santa Cruz Biotechnology, Inc.), rabbit polyclonal anti-GFP alexafluoro488 (1:1,000) (Invitrogen, Carlsbad, CA), rabbit polyclonal anti-VSV-G (1:1,000) (kindly gifted from Prof Nakamura, Kyoto Sangyo University), mouse monoclonal anti-GM130 (1:1,000) (BD transduction, San Diego, CA), mouse monoclonal anti-β-actin (1:2,000) (Sigma-Aldrich Inc., St. Louis, MO), rabbit polyclonal anti-lamin A (1:200) (Sigma-Aldrich Inc.), rabbit polyclonal anti-Thy1 (1:1,000) (Cell Signaling), rabbit monoclonal anti-GluR3 (D47E3) (1:1,000) (Cell Signaling), mouse monoclonal anti-NR1 (CT) (1:500) (Millipore Corp., Billerica, MA), mouse monoclonal anti-PrP (SAF32) (1:1,000) (Bertin Pharma, Montigny le Bretonneux, France), mouse monoclonal anti-PrP (SAF83) (1:1,000) (Bertin Pharma), mouse monoclonal anti-PrP (3F4) (1:1,000 for IHC, 1:2,000 for WB) and (6D11) (1:3,000) (Covance), mouse monoclonal 132 anti-PrP (1:10,000) (mAb132, kindly gifted from Prof Horiuchi, Hokkaido University), goat anti-mouse IgG AlexaFluoro488 (1:2,000) (Molecular Probes, Eugene, OR), goat anti-rabbit IgG Cy3 (1:1,000) (Amersham Biosciences Inc., Piscataway, NJ), goat anti-mouse IgG horseradish peroxidase (HRP) (1:3,000) (GE Healthcare, Little Chalfont, UK), goat anti-rabbit IgG HRP (1:3,000) (GE Healthcare) and DyLight 649 donkey anti-rabbit IgG minimal X-reactivity Ab (1:1,000) (Biolegend, San Diego, CA). 4′,6-Diamidino-2-phenylindole (DAPI) was purchased from Sigma-Aldrich. Sulfo-NHS-LC-Biotin and NeutrAvidin UltraLink Resin were purchased from Thermo Scientific (Rockford, IL). Cell lines N2aC24, N2aC24L1-3 and N2aC24Chm cells were established elsewhere [23] . N2a cells (ATCC CCL-131, kindly gifted from Prof Horiuchi, Hokkaido University) were permanently transfected with pEF1/Myc-His A (Invitrogen) encoding mouse PrP C . N2aC24 cells were subsequently cloned from among G418-resistant colonies. N2aC24L1-3 and N2aC24Chm cells were obtained by limiting dilution of N2aC24 cells exposed to 22L and Chandler scrapie [42] . Cured N2aC24L1-3 and N2aC24Chm cells were established by incubation with anti-PrP SAF32 Ab at 2–4 μg ml −1 . Cells were tested for PrP Sc by WB and if it was undetectable, they were maintained in the media minus Ab with occasional checks for PrP Sc . ScN2a cells were a gift from Prof Doh-ura, Tohoku University. Cells were maintained at 37 °C with 5% CO 2 in air in Dulbecco’s Modified Eagle Medium (Invitrogen) containing 10% fetal bovine serum (FBS). WB analysis Cells or brain tissues were lysed in lysis buffer (150 mM NaCl, 50 mM Tris–HCl (pH 7.5), 0.5% Triton X-100, 0.5% sodium deoxycholate, 1 mM EDTA) containing protease inhibitor cocktail (Nakalai Tesque Co., Kyoto, Japan), and protein concentration was measured by BCA assay kit (Pierce, Rockford, USA). Total proteins were treated with PK (20 μg mg −1 total proteins) at 37 °C for 30 min. PK was inactivated by heating at 99 °C for 10 min in Laemmli’s sample buffer. The samples were loaded into a SDS–polyacrylamide gel. After electrophoresis, proteins were electrotransferred onto an Immobilon-P PVDF membrane (Millipore Corp.). The membrane was blocked in 5% skim milk in PBS containing 0.1% Tween 20 and incubated with first Ab followed by horseradish peroxidase-conjugated secondary Ab. Signals were visualized using Immobilon Western Chemiluminesent HRP substrate (Millipore Corp.) and detected by LAS-4000 mini (Fujifilm Co., Tokyo, Japan). Biotinylation of cell surface proteins Cells (85–95% confluent) were washed with PBS three times and incubated with 2 ml of 1 mg ml −1 Sulfo-NHS-LC Biotin (Thermo Scientific) in PBS for 30 min at room temperature (RT). The cells were then washed with 0.1 M Glycine in PBS three times and ice-cold PBS three times and lysed in lysis buffer. Two miligrams of the total proteins were mixed with 10 μl (bed volume) of NeutrAvidin UltraLink Resin (Thermo Scientific) for 4 h at 4 °C and the biotinylated protein–resin complexes were collected by brief microcentrifugation. The complexes were then washed with the lysis buffer three times and heated at 99 °C for 10 min in 40 μl of Laemmli’s sample buffer to separate the biotinylated proteins from the complexes. The biotinylated proteins in the supernatant were subjected to WB. For biotinylation of surface proteins in the brain tissues, brains were removed from terminally ill male ICR mice (Charles River Laboratories, Kanagawa, Japan) infected with RML and 22L scrapie prions and from PBS-inoculated age-matched male ICR mice simultaneously, immediately sectioned into 1.5-mm-thick segments using a mouse brain slicer (MB-SSC.5-C, Muromachi Kikai, Tokyo, Japan), and then soaked in 1 mg ml −1 Sulfo-NHS-LC Biotin in PBS (pH 8.0) with gentle mixing at 4 °C overnight. The brain slices were washed with 0.1 M glycine in ice-cold PBS and then PBS only three times each, and homogenized in lysis buffer. Three milligrams of the total proteins were then mixed with 20 μl (bed volume) of NeutrAvidin UltraLink Resin (Thermo Scientific) for 4 h at 4 °C. Other subsequent procedures are as described above. Immunofluorescence analysis Cells on coverslips were fixed in 3% paraformaldehyde for 15 min, treated with 0.1 M glycine in PBS for 10 min and permeabilized with 0.1% Triton X-100 in PBS for 4 min at RT. To detect PrP Sc , the cells were treated with 5 M guanidinium thiocyanate for 10 min at RT [25] . After washing with PBS, the cells were incubated with the first Ab in 5% FBS in PBS and then with fluorescent secondary Ab. After washing, the coverslips were mounted with Prolong Gold antifade reagent (Invitrogen). Fluorescent images were visualized using BIOREVO BZ-9000 (Keyence, Osaka, Japan) and fluorescent intensity was analysed using a BZ-II analyzer (Keyence). VSV-G(ts045)–GFP transport assay Cells were transfected with a vector encoding VSV-G(ts045)–GFP [43] (kindly gifted from Prof Nakayama, Kyoto University) using Lipofectamine 2000 reagent (Invitrogen) and incubated at the non-permissive temperature of 39.5 °C for 16 h to allow accumulation of VSV-G(ts045)–GFP in the ER [44] . The cells were then cultured at the permissive temperature of 32 °C in the presence of 100 μg ml −1 cycloheximide to induce transport of the already synthesized VSV-G(ts045)–GFP from the ER to the plasma membrane via the Golgi apparatus. The cells were fixed with 3% paraformaldehyde at various time points after the cell culture commenced at 32 °C, permeabilized with 0.1% Triton X-100 in PBS and stained for VSV-G(ts045)–GFP using anti-GFP Ab. The Golgi apparatus and the nucleus were also stained using anti-GM130 Ab and DAPI, respectively. The fluorescent intensities of VSV-G(ts045)–GFP in the Golgi area, which was defined as a GM130-positive area, were measured as described above from randomly selected 14–16 cell fields at each time point. The fluorescent intensities of VSV-G(ts045)–GFP in the whole cells were also measured. Trafficking of VSV-G(ts045)–GFP in the cells was assessed as the kinetics of the protein in the GM130-positive Golgi area. The kinetics was defined as a change in the ratio of the fluorescent intensities of VSV-G(ts045)–GFP in the Golgi area to those in the whole cell over time. FACS analysis of VSV-G(ts045)–GFP transport Cells transiently transfected with the VSV-G(ts045)–GFP vector were cultured at 32 °C for 0 or 120 min with 100 μg ml −1 cycloheximide after being cultured at 39.5 °C for 16 h. The cells were then washed with ice-cold PBS three times and removed by pipetting. The cells were blocked by incubation at 4 °C for 30 min with 5% FBS in PBS. The cell surface VSV-G(ts045)–GFP was labelled with anti-VSV-G Ab (a gift from Prof Nakamura, Kyoto Sangyo University) at 4 °C for 1 h in 5% FBS-containing PBS without detergents. After three washes with ice-cold PBS, the cells were reacted with DyLight 649 donkey anti-rabbit IgG minimal X-reactivity Ab (Biolegend, San Diego, CA) at 4 °C for 1 h in 5% FBS-containing PBS. The cells were then washed three times with ice-cold PBS, resuspended in 1 ml of ice-cold PBS and analysed by FACS. Insulin stimulation Cells were washed with and incubated with KRH buffer (20 mM HEPES (pH 7.4), 136 mM NaCl, 4.7 mM KCl, 1.25 mM MgSO 4 , 1.25 mM CaCl 2 ) containing 0.1% (w/v) bovine serum albumin for 1 h at 37 °C. Insulin was then added at a final concentration of 10 −7 M for 10 min. After washing with ice-cold PBS three times, the cells were lysed in lysis buffer containing 5 mM sodium vanadate, 10 mM β-glycerophosphate and 5 mM sodium molybdate, and subjected to WB. Transfection Cells were transiently transfected with pcDNA3.1 expression vectors (Invitrogen) encoding hamster or human PrP C using Lipofectamine 2000 reagent (Invitrogen). The cells were lysed in lysis buffer 2 days after transfection and subjected to WB. Statistical analysis Data were analysed using the Student’s t -test. How to cite this article: Uchiyama, K. et al . Prions disturb post-Golgi trafficking of membrane proteins. Nat. Commun. 4:1846 doi: 10.1038/ncomms2873 (2013).